Asymmetric spermatocyte division as a mechanism for controlling sex ratios Although Mendel's first law predicts that crosses between XY (or XO) males and XX females should yield equal numbers of males and females, individuals in a wide variety of metazoans transmit their sex chromosomes unequally and produce broods with highly skewed sex ratios. Here, we report two modifications to the cellular programme of spermatogenesis, which, in combination, help to explain why males of the free-living nematode species Rhabditis sp. SB347 sire <5% male progeny. First, the spermatogenesis programme involves a modified meiosis in which chromatids of the unpaired X chromosome separate prematurely, in meiosis I. Second, during anaphase II, cellular components essential for sperm motility are partitioned almost exclusively to the X-bearing sperm. Our studies reveal a novel cellular mechanism for the differential transmission of X-bearing sperm and suggest Rhabditis sp. SB347 as a useful model for studying sex chromosome drive and the evolution of new mating systems. Just as Mendel's first law predicts that crosses between XY (or XO) males and XX females should yield a 1:1 ratio of males and females, standard models in population genetics predict that the most evolutionarily stable strategy for sexually reproducing organisms is to produce equal proportions of sexes [1] , [2] . Selection forces are predicted to favour parents that invest equal resources to offspring of both sexes, as deviations from this equality would immediately result in counterbalancing selection favouring the underrepresented sex [1] , [3] . However, certain ecological and genetic conditions may violate these assumptions, resulting in sex ratios that depart significantly from 50% (ref. 4 ). Theoretical models of how individuals should optimally allocate resources to male or female reproduction, termed sex allocation, predict that female biased sex ratios are favoured when mating competition occurs primarily between brothers and close relatives [5] , [6] . Consistent with these theories, individuals, in a wide variety of metazoans, have been reported to transmit their sex chromosomes unequally and produce broods with highly skewed sex ratios. In genetic crosses, distorted sex ratios within individual broods are proposed to occur in one of three ways [7] : nonrandom segregation of a sex chromosome during the meiotic divisions [8] , sex chromosome specific differences in sperm function due to differences in post-meiotic gene expression in the haploid gametes [9] or post-zygotic mechanisms that result in sex-specific embryonic lethality [10] , [11] . Yet, with the exception of recent studies of X-chromosome drive in Drosophila [12] , relatively little is known about the underlying molecular and cellular mechanisms of sex ratio distortion. As a large and evolutionary deep phylum, nematodes are a promising group in which to study sex ratio distortions. Although many nematodes exist as male/female species, the phylum as a whole exhibits a large diversity of reproductive systems ranging from male/female systems to hermaphroditism and parthenogenesis [13] . Nematodes are also ecologically diverse as they fill multiple niches as both ubiquitous members of the meiofauna and are parasites of agricultural and medical consequence. As a result, males in closely related species often experience dramatically different levels of sperm competition [14] . High levels of sperm competition have been associated with increased sperm size [14] ; and, at least in Caenorhabditis briggsae , selection for X-bearing male sperm that are more competitive than non-X-bearing male sperm [15] . Importantly, many parasitic nematodes exhibit striking skewed sex ratios that are proposed to be adaptive to their specific environmental conditions and lifecycles. For example, mostly or exclusively feminine broods have been reported in male–female crosses of both the insect parasite Heterorhabditis [16] and the rat parasite Strongyloides ratti [17] . However, as genetic studies of parasitic nematodes can be challenging, the recent discovery that males in the free-living nematode species, Rhabditis sp. SB347 sire almost exclusively progeny of the feminine sex, suggests that this species that can be cultured in the laboratory might be ideal for investigating the cellular basis of sex chromosome drive [18] . Here, we report a novel mechanism for pre-zygotic sex ratio distortion that helps to explain why males of the free-living nematode species Rhabditis sp. SB347 sire <5% male cross-progeny. First, a modified meiotic programme in males enables the sister chromatids of the unpaired X chromosome to separate equationally during meiosis I, and thus shifts the asymmetric reductive division of the X chromosome to meiosis II. Second, during anaphase II, the meiotic spindle becomes highly asymmetric with a dominant pole on the X-bearing side, a morphology that correlates with the cellular components essential for sperm viability and motility being partitioned almost exclusively to the X-bearing sperm. In favouring transmission of X-bearing sperm, Rhabditis sp. SB347 males produce an excess of daughters, a reproductive strategy that is predicted to maximize the reproductive output in a species that includes self-fertile hermaphrodites and colonizes ephemeral nutrient- and bacteria-rich environments. Testing alternative models of sex-ratio distortion Similar to the extensively studied nematode Caenorhabditis elegans and most other free-living nematodes, Rhabditis sp. SB347 has two sexes that are determined by an XX:XO mechanism [13] , [19] (see below). However, although C. elegans males sire equal numbers of XX hermaphrodite and XO male progeny, Rhabditis sp. SB347 males mated to females were reported to sire only 4 out of 253 (1.6%) male progeny, suggesting a highly preferential transmission of the X chromosome [18] . Our own crosses between males and females resulted in similar low proportions of male offspring (median=2.3%, n =complete broods from 24 crosses). To further character the nature of the sex ratio distortion, we tested two alternative models: differential sperm competition and differential post-zygotic lethality. In the nematode C. briggsae , X-bearing male sperm have been shown to have a competitive advantage over non-X-bearing male sperm, resulting in the production of a higher proportion of XX hermaphrodites in the first 24 h after fertilization [15] . However, when we similarly monitored the broods from eight male/female crosses of Rhabditis sp. SB347, we failed to observe dramatic shifts in the percentage of males over time ( Fig. 1 ). These results suggest that sex ratio distortion is not due to preferential fertilization by the X-bearing sperm, but rather to the near absence of functional nullo-X sperm. Likewise, when we monitored embryonic and larval viability for evidence of post-zygotic lethality, we found no evidence of either dying embryos or dead larvae ( n >80 broods). 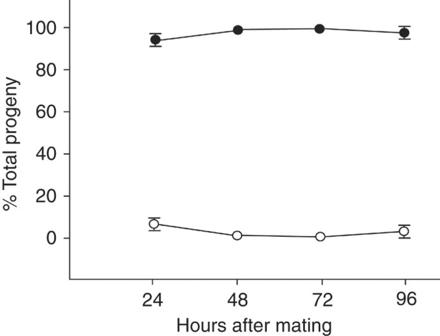Figure 1: Test for potential sperm competition. Mean percentage of outcross progeny produced by eight mated females as a function of time after mating. The proportion of F1 males (open circles) over time compared with the proportion of the feminine sex (females+hermaphrodites; filled circles). (Error bars=s.e.m.;n=8, where none are visible, the error is smaller than the symbol.) Figure 1: Test for potential sperm competition. Mean percentage of outcross progeny produced by eight mated females as a function of time after mating. The proportion of F1 males (open circles) over time compared with the proportion of the feminine sex (females+hermaphrodites; filled circles). (Error bars=s.e.m. ; n =8, where none are visible, the error is smaller than the symbol.) Full size image Interestingly, the XX sex of Rhabditis sp. SB347 includes two sexual morphs: true females and highly dispersive, self-fertilizing hermaphrodites [18] . To determine whether the anti-male skew could be generalized to these two distinctive feminine sexual morphs, we examined broods from males crossed to sperm-depleted hermaphrodites. However, we detected no statistically significant differences in male proportions ( U =378, z =−1.3, not significant) between the F1 progeny from females ( n =24 broods) and sperm-depleted hermaphrodites ( n =39 broods). Noncanonical patterns of meiotic chromosome segregation To investigate the underlying cause of the distorted sex ratio from a different perspective, we examined the cytology of spermatogenesis in Rhabditis sp . SB347 males. Using a combination of differential interference contrast (DIC) optics and the fluorescent DNA dye, Hoechst 33342, our analysis of meiotically dividing spermatocytes revealed that the larger C. elegans and smaller Rhabditis sp. SB347 male spermatocytes differed in two ways ( Fig. 2 ). First, the males differ in how they segregate their unpaired X chromosome during meiosis ( Fig. 2b ). During meiosis I, the unpaired X in C. elegans spermatocytes routinely 'lags' as it segregates to one of the two secondary spermatocytes [20] , [21] . During meiosis II, only one secondary spermatocyte possesses an X, and the sister chromatids of this X segregate equationally to its two daughter spermatids. In Rhabditis sp. SB347, we never observed a lagging chromosome during meiosis I. Yet, during meiosis II, we almost always observed a lagging chromosome segregating unequally to one of the two spermatids. Presuming that, as in other nematode studies, this lagging chromosome is the unpaired X, these results suggest that the unpaired X precociously splits into sister chromatids during meiosis I, leaving the lone X chromatid to segregate reductionally during meiosis II (summarized in Fig. 2b,d ). Therefore, we will hereafter refer to this lagging chromosome as the X, and the spermatids with the larger chromatin mass as the X-bearing spermatids. 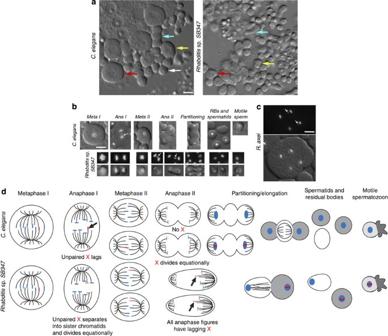Figure 2: Comparison of male spermatogenesis inC. elegansandRhabditissp. SB347. (a) Relative sizes of spermatocytes and sperm in monolayer preparations from isolatedC. elegansandRhabditissp. SB347 male gonads. Arrows indicate examples of a primary spermatocyte (red), secondary spermatocyte (yellow), the partitioning process following anaphase II (blue) and a haploid spermatid (white). (b) Comparison of the meiotic divisions and post-meiotic programme ofC. elegansandRhabditissp. SB347 spermatocytes as viewed under differential interference contrast (DIC) optics and DNA stained by Hoechst 33342. Arrows indicate a lagging X chromosome during anaphase I inC. elegansand similar lagging chromosomes during anaphase II inRhabditissp. SB347. DuringC. elegansspermatogenesis, cellular components that are no longer needed partition into a central residual body (RB), which appears smooth under DIC optics (partitioning). During the partitioning stage inRhabditissp. SB347, no residual bodies form, but one spermatid (on the left in these images) appears smooth relative to the other. As in other nematodes, the motile spermatozoa lack flagella and instead crawl using a pseudopod.Meta I, metaphase I;Ana I, anaphase I;Meta II, metaphase II;Ana II, anaphase II. (c) Anaphase II spermatocytes fromR. axeishowing lagging Xs (arrows) in sister secondary spermatocytes. Because of flattening, the partial cleavage furrows have regressed. (d) Schematic diagram showing the differential segregation pattern of the known (and presumed) X chromosome (marked in red) and the distinct post-meiotic morphology changes. In meiosis I, the unpaired X segregates either reductively (C. elegans) or equationally (Rhabditissp. SB347). During meiosis II, the single X chromatid inRhabditissp. SB347 secondary spermatocytes segregates reductively to one of the two spermatids. During post-meiotic partitioning, essential cellular components (grey) are segregated to the future spermatozoan while nonessential materials (white) are segregated to either the residual body (C. elegans) or the non-X sperm (Rhabditissp. SB347). Microtubules are indicated by black lines. All images ina–care at the same scale; scale bar, 5 μm. Figure 2: Comparison of male spermatogenesis in C. elegans and Rhabditis sp. SB347. ( a ) Relative sizes of spermatocytes and sperm in monolayer preparations from isolated C. elegans and Rhabditis sp. SB347 male gonads. Arrows indicate examples of a primary spermatocyte (red), secondary spermatocyte (yellow), the partitioning process following anaphase II (blue) and a haploid spermatid (white). ( b ) Comparison of the meiotic divisions and post-meiotic programme of C. elegans and Rhabditis sp. SB347 spermatocytes as viewed under differential interference contrast (DIC) optics and DNA stained by Hoechst 33342. Arrows indicate a lagging X chromosome during anaphase I in C. elegans and similar lagging chromosomes during anaphase II in Rhabditis sp. SB347. During C. elegans spermatogenesis, cellular components that are no longer needed partition into a central residual body (RB), which appears smooth under DIC optics (partitioning). During the partitioning stage in Rhabditis sp. SB347, no residual bodies form, but one spermatid (on the left in these images) appears smooth relative to the other. As in other nematodes, the motile spermatozoa lack flagella and instead crawl using a pseudopod. Meta I , metaphase I; Ana I , anaphase I; Meta II , metaphase II; Ana II , anaphase II. ( c ) Anaphase II spermatocytes from R. axei showing lagging Xs (arrows) in sister secondary spermatocytes. Because of flattening, the partial cleavage furrows have regressed. ( d ) Schematic diagram showing the differential segregation pattern of the known (and presumed) X chromosome (marked in red) and the distinct post-meiotic morphology changes. In meiosis I, the unpaired X segregates either reductively ( C. elegans ) or equationally ( Rhabditis sp. SB347). During meiosis II, the single X chromatid in Rhabditis sp. SB347 secondary spermatocytes segregates reductively to one of the two spermatids. During post-meiotic partitioning, essential cellular components (grey) are segregated to the future spermatozoan while nonessential materials (white) are segregated to either the residual body ( C. elegans ) or the non-X sperm ( Rhabditis sp. SB347). Microtubules are indicated by black lines. All images in a – c are at the same scale; scale bar, 5 μm. Full size image To determine whether this noncanonical pattern of X-chromosome segregation was sufficient to explain the distorted sex ratio, we also examined spermatogenesis in the closely related male–female species Rhabditella axei [22] . However, despite having a 1:1 sex ratio, spermatocytes in R. axei and at least some other nematode species [23] also exhibit a similar noncanonical pattern of X-chromosome segregation with lagging Xs routinely observed in anaphase II spermatocytes ( Fig. 2c ). Therefore, this atypical meiotic pattern alone is insufficient to explain the distorted sex ratio in Rhabditis sp. SB347. Essential components partition to X-bearing spermatids A second major difference between male spermatogenesis in C. elegans and Rhabditis sp. SB347 involves the morphological changes and cytoplasmic partitioning events that follow anaphase II. In C. elegans spermatocytes, anaphase II is followed by an asymmetric partitioning event during which cellular components not required for spermatozoan function are selectively partitioned for disposal into a central residual body. In C. elegans , this partitioning process requires myosin VI (ref. 24 ) and is accompanied by dynamic changes in both actin and microtubule superstructures, both of which ultimately partition to the residual body [25] ( Fig. 2b,d ). In Rhabditis sp. SB347 male spermatocytes, anaphase II is followed by an elongation phase during which the putative X-bearing spermatid receives most of the optically refractive material ( Fig. 2b,d ). In contrast, the nullo-X spermatid appears notably 'smoother' under DIC optics and similar to the 'smooth' residual bodies in C. elegans ( Fig. 2b ). To further investigate this asymmetric partitioning event and the refractive material that segregates to the putative X-bearing spermatids, sperm monolayers from Rhabditis sp. SB347 males were immunostained with antibodies against the major sperm protein (MSP). During C. elegans spermatogenesis, MSP exhibits a predictable localization pattern: as MSP is synthesized, it initially assembles into fibrous bodies within developing spermatocytes; then, following anaphase II, these MSP fibrous bodies segregate specifically to the spermatids and away from the residual body before the fibrosis bodies disassemble and MSP distributes throughout the spermatid cytoplasm. Later, during sperm activation, MSP localizes to the pseudopod where it serves as the major motility protein of the crawling spermatozoan [26] . During Rhabditis sp. SB347 spermatogenesis, these MSP-rich fibrous bodies distributed equally to the secondary spermatocytes during the first meiotic division, but following anaphase II, they almost always segregated specifically to the X-bearing spermatid ( Fig. 3a ). In a complementary manner, actin, which normally partitions to the residual body in C. elegans [27] , partitioned predominantly to the nullo-X spermatid in Rhabditis sp. SB347, although small amounts of actin often remained detectable around the chromatin mass of the X-bearing sperm ( Fig. 3b,c ). As MSP is absolutely essential for nematode sperm motility, these results suggest that these nullo-X spermatids assume the disposal function of residual bodies and that only the X-bearing spermatids retain the capacity to mature into motile spermatozoa. 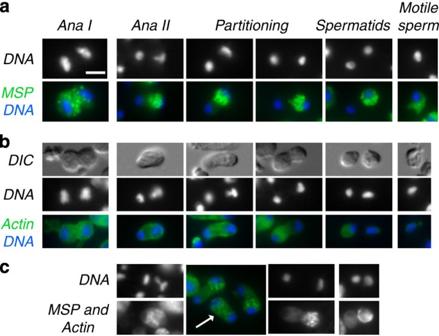Figure 3: Differential partitioning of cellular components following anaphase II. (a) Localization and partitioning of the major sperm protein (MSP) relative to the stage of spermatogenesis. Immunostaining of MSP (green), 4,6-diamidino-2-phenylindole (DAPI)-stained DNA (white or blue). During the meiotic division and the partitioning process, MSP localizes to punctuate fibrosis bodies. In motile spermatozoa, MSP localizes uniformly throughout the pseudopod but is absent in the cell body.Ana I, anaphase I;Ana II, anaphase II. (b) Localization and partitioning of actin (green) to the sperm with the smaller chromatin mass DNA (white or blue). (c) In co-stained cells, using a single anti-mouse secondary antibody, the punctuate MSP fibrosis bodies partition to the sperm with the X and the larger chromatin mass, whereas the smooth and less intense actin staining pattern is associated with the other spermatid. Arrow points to a rare instance of symmetric MSP partitioning. All images are at the same scale; scale bar, 3 μm. Figure 3: Differential partitioning of cellular components following anaphase II. ( a ) Localization and partitioning of the major sperm protein (MSP) relative to the stage of spermatogenesis. Immunostaining of MSP (green), 4,6-diamidino-2-phenylindole (DAPI)-stained DNA (white or blue). During the meiotic division and the partitioning process, MSP localizes to punctuate fibrosis bodies. In motile spermatozoa, MSP localizes uniformly throughout the pseudopod but is absent in the cell body. Ana I , anaphase I; Ana II , anaphase II. ( b ) Localization and partitioning of actin (green) to the sperm with the smaller chromatin mass DNA (white or blue). ( c ) In co-stained cells, using a single anti-mouse secondary antibody, the punctuate MSP fibrosis bodies partition to the sperm with the X and the larger chromatin mass, whereas the smooth and less intense actin staining pattern is associated with the other spermatid. Arrow points to a rare instance of symmetric MSP partitioning. All images are at the same scale; scale bar, 3 μm. Full size image Meiotic spindles become asymmetric during anaphase II As asymmetries in the number and/or the size of centrosomes have the potential to distort the symmetry of the microtubule spindle [7] , we wondered whether the lagging chromosome in Rhabditis sp. SB347 spermatocytes might bias the partitioning of MSP fibrous bodies through a microtubule mediated process. To test this hypothesis, we examined the morphology of the microtubule spindles ( Fig. 4 ). During both metaphase I and II, the spindles were symmetric. However, beginning in anaphase II, the spindles became increasingly asymmetric as microtubules accumulated at the putative X-bearing pole. This spindle asymmetry coupled with the small size of the Rhabditis sp. SB347 spermatocytes and the close temporal association of post-meiotic residual body formation seems to strongly bias the partitioning of MSP fibrous bodies towards the X-bearing sperm. Consistent with this model, partitioning of C. elegans fibrous bodies also occurs while the microtubules are in an anaphase II configuration [21] , [28] , [29] . Only later do the microtubules disassociate from the chromatin masses and move centrally into either the residual body ( C. elegans ) or the nullo-X spermatid ( Rhabditis sp. SB347). 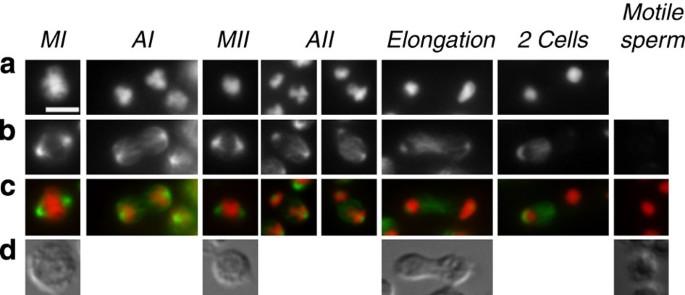Figure 4: Microtubule dynamics during and following the meiotic divisions. (a–c) In methanol fixed sperm spreads, DNA was labelled with DAPI (a) and tubulin was labelled with FITC-conjugated anti-α-tubulin monoclonal DM14 (Sigma) (b). In the merge image (c), DNA is red and tubulin is green. Spindles are symmetric during metaphase I and II, but become biased towards the X-chromosome side during anaphase II. During the elongation stage, microtubules reposition to the spermatid that has the smaller chromatin mass. (d) DIC images. All images are at the same scale; scale bar, 3 μm.MI, metaphase I;AI, anaphase I;MII, metaphase II;All, anaphase II. Figure 4: Microtubule dynamics during and following the meiotic divisions. ( a – c ) In methanol fixed sperm spreads, DNA was labelled with DAPI ( a ) and tubulin was labelled with FITC-conjugated anti-α-tubulin monoclonal DM14 (Sigma) ( b ). In the merge image ( c ), DNA is red and tubulin is green. Spindles are symmetric during metaphase I and II, but become biased towards the X-chromosome side during anaphase II. During the elongation stage, microtubules reposition to the spermatid that has the smaller chromatin mass. ( d ) DIC images. All images are at the same scale; scale bar, 3 μm. MI , metaphase I; AI , anaphase I; MII , metaphase II; All , anaphase II. Full size image Together, our findings indicate that the production of excess feminine progeny by Rhabditis sp. SB347 males reflects the near absence of putative nullo-X sperm among their motile spermatozoa. Furthermore, our data suggest a three-step process to account for the observed bias ( Fig. 2d ). First, the disassociation of the putative unpaired X into sister chromatids during meiosis I shifts the reductive division of the X-chromosome to meiosis II. Second, this X-chromosome asymmetry, potentially in conjunction with the small size of the Rhabditis sp. SB347 spermatocytes, triggers an accumulation of microtubules at the X-bearing pole. Last, the resulting microtubule asymmetry coupled with the close temporal association of post-meiotic residual body formation strongly biases MSP partitioning into the X-bearing sperm. The actual partitioning process is likely to involve the same microtubule and actin/myosin forces that are proposed to partition residual body components from haploid nematode spermatids. Although we did observe rare instances of symmetric partitioning of MSP to sister spermatids ( Fig. 3c ), the extreme consistency and efficiency of the asymmetric partitioning raises the question of how Rhabditis sp. SB347 males sire any male progeny. We currently favour two possible models: Either the sister chromatids of the X-chromosome may occasionally fail to disassociate until meiosis II or the asymmetric X during meiosis II may occasionally fail to trigger an asymmetric partitioning event. Both models remain plausible as the timing of X-chromosome disjunction appears to be a variable trait within nematodes, and our studies of R. axei indicate that an equational division of the unpaired X during meiosis I is insufficient to bias sperm functionality. Importantly, as this particular mechanism of biasing sex ratios involves the highly conserved machinery of cell division, similar mechanisms may underlie other examples of sex chromosome drive [30] , [31] . Although further studies are required to determine the molecular details of the asymmetric division in Rhabditis sp. SB347, this study is one of the few to document, at a cellular level, how an asymmetric partitioning process can generate gametes of distinct functionality. At an evolutionary level, unequal sex ratios may be commonly favoured in nematodes, especially in hermaphroditic terrestrial free-living nematode species that colonize ephemeral nutrient- and bacteria-rich environments [32] , [33] . In species that typically reproduce in large numbers, rapidly deplete food sources, and produce highly dispersive dauer larvae; sibling matings are frequently more common than outcrossing and therefore assumptions of random matings become invalid [1] , [4] . Under these conditions, females producing 1:1 sex ratios are predicted to be at a selective disadvantage relative to those producing excess daughters [4] . These ecological conditions might also favour the evolution of X-chromosome drive, an outcome that often leads dioecious species to extinction. It is tempting to speculate that in the presence of these same pressures, Rhabditis sp. SB347 and other species have escaped extinction by evolving the ability to self-fertilize. Sex ratios Worms at the fourth larval stage were picked to single plates and sexed once they became adults. Hermaphrodites were distinguished from females by their ability to produce progeny in the absence of a mating partner. To perform crosses, hermaphrodites were first sperm-depleted by letting them self-fertilize until no more progeny was produced ( ∼ about 3 days into adulthood). A total of 1,148 F1 progeny from 24 broods were sexed for the female versus male crosses and 658 F1 progeny from 39 broods were scored for the sperm-depleted hermaphrodite versus male crosses. In all cases, broods were scored until females and hermaphrodites stopped laying eggs. In several broods, we observed discrepancies between the embryo and adult counts, which mostly likely reflect the escape of larval hermaphrodites during their dispersive (dauer) stage. As a result, our calculations of male sex ratios include only broods in which <10% of the worms were lost between the embryo and adult stages. Because male proportions of the hermaphrodite versus male crosses were not normally distributed W (39)=0.8, P <0.05), we used the nonparametric Mann–Whitney U -test for comparing male proportions. Sperm competition experiments Single Rhabditis sp. SB347 females were mated to 2–3 males for a 3-h interval. The mated females were transferred at regular intervals to fresh plates until they stopped laying eggs or died. Eggs from eight different broods were allowed to hatch and the gender of emergent worms was scored once they became adults. The numbers of resulting hermaphrodites and females were pooled and assigned as the 'feminine' sex. Immunohistochemistry and microscopy Meiotic sperm spreads for Hoechst/DIC analysis and methanol-fixed, immunofluorescence preparations were carried out as previously described [34] , [21] . In brief, male gonads were dissected in 5 μl of sperm salts on ColorFrost Plus slides (Fisher Scientific), and then a coverslip with four corner dots of silicone grease was placed over the isolated gonad and gentle pressure was used to generate a monolayer of spermatocytes and spermatids. For DIC/Hoechst studies, Hoechst 33342 (Sigma-Aldrich) was included at 100 μg ml −1 . Alternatively, the slide preparations were quick frozen in liquid nitrogen, the coverslip was removed, and the specimens were fixed overnight in −20 °C methanol. Slides were washed in PBS and blocked in PBS plus 0.5% BSA. Incubations with primary and secondary antibodies were carried out in a room temperature humid chamber using the following dilutions: 1:800 mouse anti-MSP 4D5 (ref. 35 ), 1:50 mouse anti-actin C4 (Millipore), 1:100 FITC-conjugated anti-α-tubulin monoclonal DM14 (Sigma), and 1:100 goat anti-mouse FITC-labelled IgG (Jackson Immunoresearch Laboratories). Slides were prepared with GelMount (Biomedia Corp.) as a combined mounting and anti-fade media. Images were acquired on an Olympus BX60 microscope equipped with a Cooke Sensicam and processed with IPLab or Photoshop software. For each of the figures, the composite images are based on observations of sperm spread from >60 individual males. The cytology of the various stages was highly uniform both within single male gonads and between individual males. How to cite this article: Shakes, D. C. et al . Asymmetric spermatocyte division as a mechanism for controlling sex ratios. Nat. Commun. 2:157 doi: 10.1038/ncomms1160 (2011).